Core clock genes adjust growth cessation time to day-night switches in poplar Poplar trees use photoperiod as a precise seasonal indicator, synchronizing plant phenology with the environment. Daylength cue determines FLOWERING LOCUS T 2 ( FT2 ) daily expression, crucial for shoot apex development and establishment of the annual growing period. However, limited evidence exists for the molecular factors controlling FT2 transcription and the conservation with the photoperiodic control of Arabidopsis flowering. We demonstrate that FT2 expression mediates growth cessation response quantitatively, and we provide a minimal data-driven model linking core clock genes to FT2 daily levels. GIGANTEA ( GI ) emerges as a critical inducer of the FT2 activation window, time-bound by TIMING OF CAB EXPRESSION ( TOC1 ) and LATE ELONGATED HYPOCOTYL ( LHY2 ) repressions. CRISPR/Cas9 loss-of-function lines validate these roles, identifying TOC1 as a long-sought FT2 repressor. Additionally, model simulations predict that FT2 downregulation upon daylength shortening results from a progressive narrowing of this activation window, driven by the phase shift observed in the preceding clock genes. This circadian-mediated mechanism enables poplar to exploit FT2 levels as an accurate daylength-meter. In boreal and temperate regions, trees undergo an annual alternation in the shoot apex between active growth and dormancy. Proper timing of growth cessation in autumn, which precedes dormancy, is crucial for their adaptation, thus synchronizing seasonal phenology with environmental permissiveness for growth. Trees like poplar rely on photoperiod as the most accurate cue to set the annual vegetative growing period, ceasing growth when the daylength falls below a threshold known as the critical daylength. Days with hours of light above the critical daylength are referred to as long-day (LD), while those below are called short-day (SD) [1] , [2] . Daylength input is perceived in leaves, and it sets the ~24 h oscillations of the circadian clock that ultimately converge to control the daily activation of photoperiodic effector FLOWERING LOCUS T 2 (FT2) (Fig. 1a ) [3] . Under LD, FT2 daily expression is essential for promoting shoot apex vegetative development, whereas the SD induces FT2 downregulation, marking the onset of growth cessation irrespective of the tree’s age [4] , [5] , [6] . Therefore, control of the annual growing period in poplar depends on the photoperiodic pathway rather than age-dependent regulators. Fig. 1: Daylength modulates the expression of FT2 and its transcriptional regulators to control poplar shoot apex growth. a Overview of leaf-localized daylength sensing mechanism that controls the transition from active growth to growth cessation in poplar. b Daily FT2 transcription in LD (circles, red) and SD (triangles, blue). Spots represent qPCR results, with means of the two biological replicates used for fitting highlighted. Dashed lines depict a polynomial spline fit. FT2 in SD was set to 1 due to nondetection. c FT2 expression measured by qPCR at ZT16 under different daylengths. Mean ± sd, n = 4 biological replicates. d Heat map of daily transcription patterns for the photoperiodic-responsive genes in LD and SD. qPCR means (b and Supplementary Fig. 2 ) normalized 0–1 per gene. FT2 in SD is shown in grey due to nondetection. b–d ZT, Zeitgeber Time in hours. e SD to LD deviation of the gene expression patterns shown in ( d ) for phase (time of maximal gene expression) shift, amplitude ratio, and daily total transcript ratio (AUC—Area Under the Curve) after Gaussian fit (Supplementary Fig. 2 ). Full size image In poplar, several photoperiodic-controlled genes have been proven to regulate FT2 transcription. LATE ELONGATED HYPOCOTYL 2 (LHY2) binds to 3’UTR of FT2 and is necessary for FT2 downregulation during nightlength extension. Accordingly, LHY2 overexpression reduces FT2 level, while LHY2 RNAi increases it, delaying poplar growth cessation [5] , [7] . A similar delay is observed in the RNAi of TIMING OF CAB EXPRESSION (TOC1 ) [7] . In Arabidopsis orthologs, toc1-1 knockout increases FT mRNA expression, accompanied by a slight phase shift of CONSTANS (CO) transcription to the daytime [8] . Moreover, TOC1 is a general transcriptional repressor that targets TGTG motifs through its CCT DNA-binding domain [9] . This intermolecular binding is stabilized forming a trimeric complex with NUCLEAR FACTOR Y subunits B and C (NF-YB/C) [10] . Interestingly, this mode of transcriptional regulation by TOC1 is analogous to the one previously described for CO activation of FT . The CCT domain of CO mediates its binding to two CORE sites—TGTG(N2-N3)ATG, sharing the TGTG sequence, in the proximal FT promoter [11] , and this is stabilized by CO/NF-Y interaction [12] , [13] , [14] . Arabidopsis TOC1 and CO were also reported to be associated in vivo [15] . Another circadian gene, GIGANTEA ( GI ), is critical for FT2 expression. GI RNAi drastically decreases FT2 in LD, triggering growth cessation. Conversely, GI overexpression upregulates FT2 , and growth cessation under SD is delayed [4] . In Arabidopsis , GI promotes daily FT transcription through two different pathways: 1) CO-mediated activation; GI enhances the induction of CO transcription [16] , and interacts with FLAVIN-BINDING, KELCH REPEAT, F-BOX 1 (FKF1), which ubiquitinates CO repressors CYCLING DOF FACTORS (CDFs) for degradation [17] . 2) CDF-mediated repression; the CDF family regulates CO and directly represses FT [18] . This GI-FKF1-CDF module seems to be conserved in poplar, where CDF overexpression leads to FT2 downregulation, advancing poplar growth cessation in SD [4] . Furthermore, GI is recruited to FT promoter regions in both Arabidopsis and poplar, pointing to direct FT regulation independent of the mentioned pathways [4] , [19] . Along with GI, CO is the key factor promoting FT in Arabidopsis. CO is a night-sensitive protein active at dusk in LD but degraded in SD due to night advance [20] . In poplar, CO orthologs CO1/2 promote FT2 , as CO1/2 RNAi reduces FT2 level and leads to early growth cessation in SD [21] . Intriguingly, a CO-independent repressor pathway dominates in poplar. The overexpression of either CO1 or CO2 does not upregulate FT2 expression under SD, unlike their homolog in Arabidopsis [22] , [23] , [24] . Despite a substantial body of evidence on individual roles of photoperiodic-responsive genes in modulating FT2 expression, significant gaps persist in understanding how the circadian clock collectively shapes FT2 regulation in response to environmental cues such as daylength. Arabidopsis provides insights into the genetic pathways regulating FT in flowering, which bears significant similarities and could potentially aid in our knowledge. Nevertheless, the extent of conservation between the two systems and phenological processes remains uncertain. Moreover, current models of the gene networks controlling flowering in Arabidopsis yield predictions that do not agree with observed FT mRNA levels after manipulating core clock genes LHY2 and TOC1, implying there are missing factors in our comprehension of FT2 regulation (Supplementary Fig. 1 ) [25] , [26] . To address and refine the current model of FT control, we used CRISPR genetics, temporal transcriptional analysis, and computer simulations in the poplar model system Populus tremula x P. alba . By comparing different daylength conditions, we reveal distinct roles for core clock components in tailoring temporal FT2 expression patterns in response to environmental signals. A minimal core system is composed of two time-shifted repressors and a general activator. Furthermore, we pinpoint mechanistic similarities and differences between Populus and Arabidopsis . FT2 and photoperiodic regulators of shoot apical growth expression patterns comparing LD with SD To investigate how FT2 expression level is regulated by daylength in poplar, we first recorded the daily expression pattern of FT2 mRNA. In LD (16 h light: 8 h dark) condition, FT2 showed a strong peak of expression at ZT16 (ZT refers to Zeitgeber Time, i.e. hours from dawn) in the intersection between day and night. Nevertheless, when exposed to SD condition (12 h light: 12 h dark), FT2 transcript could not be detected (Fig. 1b ). Furthermore, the maximal level of FT2 expression was gradually decaying as the daylength shortens (Fig. 1c ). These findings indicate that FT2 level is tightly controlled by the duration of the day. To further study a molecular mechanism behind this FT2 control by daylength, we studied the expression kinetics of core circadian photoperiodic regulators, by comparing their expression levels in SD and LD conditions after fitting their daily patterns to a Gaussian curve. We observed a significant advance >1.5 h of phase, defined as the time of maximal expression, for GI and CDF2 , followed by CO2 (1.3 h) and CO1 (0.8 h) in SD condition (Fig. 1 d, e, and Supplementary Fig. 2 ). Similarly, LHY2 transcription advanced 1.4 h, with a nearly 1.4-fold increase in its amplitude. Conversely, FKF1 showed minimal variations, like TOC1 , which slightly increased the total accumulated transcript 1.1 times. Interestingly, TOC1 appeared later than LHY2 in both conditions, preceding the FT2 expression peak in LD (Fig. 1 d, e and Supplementary Fig. 2 ). Notably, these observations contrast with results reported for Arabidopsis homologs, in which these core circadian clock genes, including TOC1 , exhibit a widespread phase advance when transitioning to SD (Supplementary Fig. 3 ) [27] . Also, unlike in Arabidopsis , poplar does not show an increase in GI level in the SD condition (Fig. 1e and Supplementary Fig. 3b ). Furthermore, when contrasting GI and TOC1 relative phases under LD, GI is expressed earlier than TOC1 in Arabidopsis , whereas this order is reversed in poplar. The phase advances described in SD keep GI preceding TOC1 expression in Arabidopsis , while in poplar, both expression patterns coincide with a phase ~ ZT8.5 (Fig. 1 d, e and Supplementary Fig. 3 ). Finally, poplar CO1/2 exhibit a significantly delayed expression phase compared to Arabidopsis CO, both in LD (~5 h later) and SD (~8 h later), displaying their maximum expression at the beginning of the day (Fig. 1d , Supplementary Figs. 2 a, b, and 3a ). CRISPR-Cas9 lines unveil the role of TOC1, GI, and LHY2 in regulating FT2 transcription To further dissect the role of the core circadian clock genes in poplar growth cessation and FT2 regulation, we characterized the CRISPR-Cas9 loss-of-function lines for LHY2 [5] , TOC1, and GI (see Supplementary Fig. 4 ). In LD condition, WT plants produced 3 young leaves at the apex (Fig. 2a ). In contrast, gi mutant fails to reach this stage of full growth and ceases growth one month after being transferred to soil in LD, a response reminiscent of ft2 knockout (Fig. 2a ). Conversely, lhy2 and toc1 trees, when compared to WT, require a shorter daylength (14 h instead of 15 h) to start reducing the activity of shoot apical growth and instead remain actively growing under SD condition (Fig. 2a ). Fig. 2: Circadian clock core genes TOC1, GI, and LHY2 regulate FT2 transcription. a Growth scores from 3 (full growth) to 0 (no growth) in LD and gradually shortening the daylength, indicated by boxes on the top, for WT (black) and loss-of-function lines of TOC1 (yellow), LHY2 (green), GI (purple), and FT2 (beige) [6] . Mean ± sd, n = 6 biological replicates. b Daily FT2 transcription in WT (upward triangles, black) compared to the knockout lines toc1 (squares, yellow), lhy2 (circles, green), and gi (downward triangles, purple) under LD condition. Spots depict qPCR results, with means of the two biological replicates used for fitting highlighted. Solid and dashed lines represent Gaussian and polynomial spline fits, respectively. c Heat map of daily transcription patterns for photoperiodic regulators in WT and toc1 , lhy2 , and gi knockouts, under LD. qPCR means ( b and Supplementary Fig. 5 ) normalized 0-1 per gene. Grey color indicates non-detection levels. d Deviation of the gene expression patterns shown in ( c ), comparing the respective knockout line to WT, for phase (time of maximal expression) shift, amplitude ratio, and daily total transcript ratio (AUC—Area Under the Curve). e Relative mRNA accumulation of FT2 , CO1 , and CO2 at ZT16 (left panel) after transiently overexpressing 35 S::TOC1 (red) or empty vector used as control (grey) in LD. Right panel shows TOC1 levels. Mean ± sd, n = 6 biological replicates. Two-sided Student’s t -test, p-values from left to right: 0.0012 (**), 0.9558 (n.s.—not significant), 0.3056 (n.s. ), and 0.0053 (**). b , c , e ZT, Zeitgeber Time in hours. Full size image This growth cessation phenology in Populus tightly correlates with FT2 expression level observed in LD condition. In gi , FT2 mRNA remains undetected, whereas in lhy2 and toc1 , there is a similar significant increase in both amplitude (up to 2.4-fold and 2.0-fold, respectively) and total daily transcript accumulation (up to 2.4-fold and 2.3-fold, respectively) compared to WT (Fig. 2b–d ). Moreover, the expression phase of FT2 is markedly advanced by 1.1 h in lhy2 and 1.5 h in toc1 mutants (Fig. 2b–d ). Regarding the daily patterns of FT2 photoperiodic regulators, in lhy2 , it is noteworthy the phase advance for GI (4.2 h), CO1 (9.2 h), CO2 (8.6 h), and CDF2 (7.0 h) (Fig. 2 c, d , and Supplementary Fig. 5 ). However, TOC1 shows a minor delay and reduction in amplitude (0.6-fold). In toc1 , there is also a phase advance, albeit less pronounced, for CO1 (1.1 h), CO2 (4.9 h), LHY2 (1.2 h), and CDF2 (1.2 h), along with a 1.7-fold increase in the amplitude of CDF2 (Fig. 2 c, d , and Supplementary Fig. 5 ). Last, in gi , we observed a remarkable overexpression of CDF2 with an amplitude increase of more than 2.1-fold and a phase advance of 7.5 h, coinciding with the peak of FT2 transcription in the WT (Fig. 2 c, d , and Supplementary Fig. 5 ). These data emphasize the central role for GI in the activation of FT2 , as well as likely redundant role of LHY2 and CDF2 in repressing FT2 once its peak of expression is established. Our data also indicate a putative role for TOC1 in repressing FT2 during the day to complement LHY2 and CDF2 action. In the current model of FT regulation, TOC1 has never been associated with daytime repression, neither in poplar nor in Arabidopsis , even though it is known to bind the common regulator occupied by CO [9] , [10] , [11] , [12] , [13] , [14] . Furthermore, we found that TOC1-CCT domains for DNA binding are conserved between both species, and we identified the putative binding sites for Arabidopsis TOC1 and CO present in poplar FT2 promoters (Supplementary Fig. 6 ). Based on this evidence, we tested whether transiently overexpressing 35S::TOC1 construct in poplar represses FT2 transcription. Remarkably, we observed a significant reduction of more than 0.6-fold in the expression of FT2 under LD, specifically at its peak of expression, with no noticeable change in the transcription of either CO1 or CO2 (Fig. 2e ). These results indicate that TOC1 represses FT2 independently of CO1/2 and likely shapes the characteristics of FT2 expression peak. A minimal computer model recapitulates experimental patterns of FT2 transcripts, both under changes in daylength and in gain- or loss-of-function mutants for TOC1, GI, and LHY2 To better understand the interaction between circadian clock elements in FT2 transcript regulation we constructed an experimental data-driven computational model. This model represents a system of Ordinary Differential Equations (ODEs) that describes relations between changes in transcripts of core clock genes and FT2 expression (See Supplementary Note 1 for model details). In particular, we intended to construct a minimal quantitative model that yields predictions directly comparable to experimental measurements. Based on experimental findings, we considered that FT2 upregulation is largely mediated by a combination of GI’s direct and indirect activation effects since it is an essential modulator of FT2 transcription (Fig. 2b ). Given the considerable time lag between GI and FT2 expression, we hypothesized a putative daytime repressor of FT2 that would prevent early FT2 transcription. TOC1 would fulfill this function by competing with the activators, such as CO-like genes, for the binding to the FT2 promoter. Additionally, we recognized the necessity of a second repressor to control FT2 expression after its peak time, and our experimental data indicates that LHY2 fits this role by repressing FT2 during the nighttime and early morning (Fig. 3a ). Fig. 3: A minimal model that incorporates circadian regulation by TOC1, GI, and LHY2 reflects FT2 transcription dynamics under changing daylengths and genetic variations. a Photoperiodic regulators and interactions controlling FT2 expression described in poplar [4] , [5] , [21] . TOC1 repressive role is suggested in this work. Circadian clock genes integrated in the model are highlighted. Green and red colors denote positive and negative regulators, respectively. b Simulated FT2 transcription fit (LD-red, SD-blue) to experimental data (spline fitted; LD-black/solid, SD-black/dashed). c Simulated FT2 expression at ZT16 (peak) under different daylengths. d Predicted FT2 expression fold change at ZT16 for indicated photoperiods (values in c ; grey bars) compared to experimentally observed (calculated from mean values shown in Fig. 1c ; white bars). e Phase expression patterns of TOC1 (red), GI (green), and LHY2 (yellow) open a window for FT2 transcription (black) in LD (top panel), which closes transitioning to SD to suppress FT2 expression (bottom panel). Gene expression is normalized to 0-1 for visualization. Related to Supplementary Fig. 8 and Supplementary Movie 1 . f– h FT2 expression predictions in simulated loss-of-function mutants for GI ( f ), TOC1 ( g ), and LHY2 ( h ) (solid lines) compared to experimental data (spline fitted; dashed lines) under LD. WT expression in black. i– k Simulated FT2 transcription after constitutive overexpression of GI ( i ), TOC1 ( j ), and LHY2 ( k ) compared to WT in LD (black/solid) and in SD (black/dashed) predictions. j For TOC1, two levels of ectopic expression were considered. See Supplementary Note 1 for details. ZT, Zeitgeber Time in hours. Full size image Our model produces a fair quantitative fit for both the experimental pattern of FT2 expression in LD and the quantitative downregulation observed after gradually shortening the daylength (Fig. 3b–d ). A similar fit was obtained when considering CDF2 instead of LHY2 as the second repressor (Supplementary Fig. 7 ), suggesting redundancy in downregulating FT2 . Model simulations also indicate that, under LD, GI phase lags behind TOC1, creating a temporal window bounded earlier by TOC1 and later by LHY2, which boosts FT2 expression towards the end of the daytime. In SD condition, GI advances its phase while TOC1 remains unchanged, causing them to be expressed simultaneously, which results in a combined inhibitory effect on FT2 upregulation. This inhibition is further reinforced by the advancement of LHY2 (Fig. 3e ). Gene expression pattern changes of clock components interpolated between LD and SD predict a progressive narrowing of the FT2 activation frame, leading to its gradual downregulation transitioning to SD, again consistent with our experimental observations (Fig. 1c and Supplementary Fig. 8 ; Supplementary Movie 1 ). Next, we evaluated the predicted FT2 expression after gain- or loss-of-function for circadian clock genes in LD regime. As experimentally observed in gi knockout, simulations predict complete suppression of FT2 due to lack of activation (Fig. 3f ), whereas GI constitutive overexpression results in a pronounced and widespread increase of FT2 throughout the entire day, as previously reported (Fig. 3i ) [4] . For toc1 mutant, our model accurately captures the upregulation and phase advance of FT2 transcription (Fig. 3g ). Conversely, simulated TOC1 overexpression downregulates FT2 , albeit to a higher extent than experimentally observed after replicating TOC1 ectopic expression level at ZT16 (Fig. 3j —yellow solid line). In fact, a 0.6-fold change for FT2 expression is achieved with a more moderate overexpression of TOC1 (Fig. 3j —yellow dashed line). Simulated LHY2 overexpression fully suppresses FT2 transcription (Fig. 3k ), while LHY2 increased expression after 4-hour night extension also represses FT2 , as experimentally reported (Supplementary Fig. 9 ) [5] . Regarding lhy2 loss-of-function, it exhibits an upregulation of FT2 as expected, but earlier than observed (Fig. 3h ). This sole discrepancy between model prediction and experimental observations can be attributed to the FT2 expression definition in the model that strongly relies on GI alone, which is significantly advanced in lhy2 mutant, coupled with the lack of any repression at that time in the simulation (Fig. 2 c, d , and Supplementary Fig. 5 ), which suggests missing factors mediating GI activation. Identifying additional FT2 transcriptional regulators, such as CO-like genes that function under natural conditions would aid in quantitatively aligning the predictions for toc1 and lhy2 mutants. Lastly, we conducted a sensitivity analysis of FT2 transcription deviation following artificial perturbations of the expression patterns of these clock genes used as input, as a proxy for potential disturbances by factors not considered in our study. These simulations confirm the opposing and competitive contribution of GI (promoting) and TOC1 (repressing) in their influence on FT2 . Additionally, they clarify the role of LHY2 in dampening the FT2 peak and preventing its expression outside its designated timeframe (Supplementary Fig. 10 ). In summary our experimental results and model predictions support that a minimal system composed of the core circadian clock genes LHY2, TOC1, and GI largely explains the key aspects of FT2 temporal dynamics in response to the photoperiodic switch. Furthermore, our findings clarify the conserved mechanism for these clock components in FT regulation as well as highlight key differences between Arabidopsis and poplar that relates to specific temporal changes in clock gene expression dynamics. Plant photoperiodic time measurement mechanism relies on the coincidence of daylength and the circadian transcriptional activation of Flowering Locus T [5] , [8] , [21] , [28] . The expression of poplar ortholog FT2 is essential to set the boundaries of the annual vegetative growing season [6] , [29] . Here, we further demonstrate that FT2 expression level mediates the growth cessation response quantitatively. The shortening of daylight positively correlates with the decrease in the FT2 peak amplitude, and these FT2 levels are inversely linked to the photoperiod sensitivity in the studied genotypes. Specifically, in ft2 and gi mutant lines where FT2 expression is undetectable, growth ceases even under growth-promoting LD condition. Conversely, in lhy2 and toc1 mutants, growth continues under SD, with higher levels of FT2 daily expression than WT (Figs. 1 c, 2 a, and b ). This photoperiod sensitivity further underscores the relevance of each circadian clock gene in regulating the daily activation of FT2 . This study identifies TOC1 as a novel repressor of FT2 expression (Fig. 2 b and e ). In Arabidopsis, FT upregulation in the toc1-1 knockout was associated with a subtle increase in CO transcription during the light hours period, when CO protein is stable [8] , [30] . Likewise, poplar toc1 mutant displayed a slight phase advance of both CO1 and CO2 compared to WT (Fig. 2 c, d , Supplementary Fig. 5a, b ). However, ectopic TOC1 overexpression, which leads to FT2 downregulation, did not alter CO1/2 mRNA levels (Fig. 2e ), raising doubts about the regulation of CO1/2 transcription by TOC1. Based on these findings, we suggest that TOC1 regulates FT2 transcription directly and propose that it acts through protein-protein competition, interfering with the binding of FT2 activators to the promoter (Supplementary Fig. 6 ) [9] , [10] , consistent with model predictions (Fig. 3 ). Although partially supported by previous reports, the proposed model of TOC1 acting through the NF-YB/C complex would require further investigation to test the validity of this scenario both in Arabidopsis and poplar. Our results confirm that LHY2 negatively impacts poplar active growth, showing a similar effect to TOC1 during growth cessation and as a repressor of FT2 transcription (Fig. 2 a and b ). Nightlength extension promptly induces LHY2 to swiftly downregulate FT2 expression, potentially via 3’UTR interaction [5] . Integrating this direct regulation predicts FT2 transcription in LD, transitioning to SD (Fig. 3a–e ), and after nightlength extension (Supplementary Fig. 9 ), supporting LHY2 direct repressive role. qPCR patterns in lhy2 mutant suggest LHY2 may also control FT2 by modulating the other clock genes. Specifically, we observed an advance of GI and a downregulation of TOC1 in LD (Fig. 2 c, d , and Supplementary Fig. 5 ). Arabidopsis orthologs exhibit cross-regulation of LHY over GI and TOC1 that, if conserved in poplar, would explain these changes [29] . GI is indispensable to promote active growth. Our quantitative results prove that gi phenocopies ft2 mutant and both experimental qPCR patterns and model predictions indicate that it is necessary for FT2 daily expression (Figs. 2 a, b, and 3f ). Moreover, our findings provide insights into its mode of action. GI was reported to act through the control of CDFs for FT2 photoperiodic activation [4] . Experimental observations show that CDF2 mRNA is strongly advanced in gi to the time of FT2 expression, which could account for FT2 repression (Fig. 2 c, d , and Supplementary Fig. 5 ). In addition, CDF2 shifts mirror GI changes both transitioning to SD and in lhy2 (Figs. 1 e, 2d , Supplementary Figs. 2 , and 5 ) [4] , [19] . In Arabidopsis , GI represses CDFs through protein degradation mediated by FKF1 [17] . Here, we show that GI affects CDF2 transcription, a link not covered in Arabidopsis . Furthermore, the absence of transcriptional response of FKF1 in poplar to changes in daylength, unlike in Arabidopsis where FKF1 phase advances under SD, suggests a minor role of FKF1 in FT2 photoperiodic control (Fig. 1 d, e , Supplementary Figs. 2 , and 3 ). Beyond CDFs regulation, the absence of FT2 expression in gi knockout (Fig. 2b ) suggests that GI also plays a key role in promoting FT2 activation, modeled as a direct effect in our work (Fig. 3a ). However, assuming that FT2 activation solely relies on GI results in an early induction in lhy2 mutant simulation (Fig. 3h ), which is inconsistent with experimental observations (Fig. 2b ). This implies the involvement of yet unknown downstream or interacting factors in mediating GI activation. Indeed, there is no evidence that GI functions as a transcription factor despite its association with specific DNA targets [4] , [19] , [31] . A priori, we might consider GI binding mediated by CO closest orthologs. Nonetheless, CO1/2 expression patterns do not explain FT2 activation in LD in poplar WT, as they are mainly transcribed at night, when the proteins are presumably non-functional (Supplementary Fig. 2a, b ) [20] . Additionally, we found that transcriptional control of CO1/2 differs from that of CO in Arabidopsis . The gi loss-of-function does not impact on CO1 nor CO2 expression in LD, which is particularly striking given the strong upregulation of CDF2 that would lead to CO1/2 repression [4] . Moreover, lhy2 knockout also advances CO1 and CO2 phases (Fig. 2 c, d , and Supplementary Fig. 5 ). In Arabidopsis , loss of LHY function leads to an analogous increase in FT expression but without affecting CO transcription, elucidating FT upregulation through CO protein stabilization [32] . These data suggest that there is an additional link between LHY2 and CO1/2 in poplar. Overall, this divergence in CO1/2 regulation may explain their limited impact on FT2 activation, with CO-independent pathways governed by GI gaining higher relevance. Poplar co1/2 knockout would confirm or refute their necessity for FT2 expression. Consequently, other CO-like proteins with conserved functional domains may mediate GI activity with more consistent expression times for FT2 activation [3] . Additionally, these could directly compete with TOC1 to shape FT2 expression. Furthermore, we cannot dismiss the participation of genes from other families, such as Gbox-binding transcription factors given the enrichment of this motif in GI targets in Arabidopsis [31] , or the potential additive effect of multiple factors, which opens up new avenues for study. The combined temporal expression dynamics of the circadian clock genes TOC1, GI, and LHY2 in response to daylength accurately explain the changes in FT2 transcription. This study establishes a minimal model comprising three components-one activator and two repressors- in which the phase shifts controlled by the photoperiod play the pivotal role. Through computational modeling, we demonstrate the viability of GI integrating the pathways that induce FT2 under LD condition. As a result, GI creates a specific time window that enables FT2 expression in LD. During the transition to SD, this window is closed earlier in the daytime by TOC1 (via GI phase advance) and later by LHY2. Assuming that both GI and LHY2 phases progressively shift as daylength shortens, we infer that under natural conditions, from the beginning of summer, the expression window of FT2 gradually narrows, leading to a continuous reduction in FT2 expression level. Eventually, FT2 reaches a lower threshold initiating growth cessation in autumn (Fig. 3e and Supplementary Fig. 8 ; Supplementary Movie 1 ). Our model exemplifies an internal coincidence clock-driven mechanism in which core clock genes control the FT2 activity window. However, clock-independent external cues could further contribute to the modulation of FT2 expression. For instance, a rapid lengthening of night extends LHY2 expression, thereby repressing FT2 (Supplementary Fig. 9 ) [5] . In addition, putative factors mediating GI activation could integrate an external coincidence mechanism akin to CO in Arabidopsis , although, as proven in this work, not necessarily. Nevertheless, our study captures the key differences and similarities between Arabidopsis and poplar. In Arabidopsis , GI precedes TOC1 expression regardless of daylength, which would block FT upregulation in LD as modeled here, indicating the requirement of CO-mediated activation. The increased expression of GI in SD would also contradict FT downregulation (Supplementary Fig. 3 ). By contrast, in poplar TOC1 is advanced with respect to GI allowing for GI-dependent FT2 upregulation. Alternatively, in SD condition, both TOC1 and GI overlap in phase leading to strong downregulation of FT2 transcripts (Fig. 1d ). This study allowed us to identify the necessary circadian regulators and interactions for daylength control of the photoperiodic effector FT2. Future research, including explicit modeling of light input and more detailed description of the interactions presented, would contribute to build a more comprehensive framework that directly link FT2 to the environmental influences. This could lead to new strategies for modulating FT2 expression to improve tree geographical adaptation and, therefore, plantation forest breeding. Plant material and growth conditions Hybrid poplar Populus tremula x alba INRA clone 717 1B4 was used as wildtype for gene expression assays and plant transformation. Poplar plantlets were cultivated in vitro in Murashige and Skoog (MS) medium 1B (pH 5.7), supplemented with 2% sucrose, indole acetic and indole butyric acids (0.5 mg/L), and 0.7% (w/v) plant agar. Plants were grown under 16 h light:8 h dark photoperiod, 21 °C, 65% humidity, and 300-350 μmol m-2 s-1 PPFD (Photosynthetic Photon Flux Density) conditions for 2 weeks. For time-course qPCR experiments, poplars were kept in vitro for an additional week under the same conditions in LD assays. Alternatively, for shorter daylengths, photoperiod was adjusted accordingly before use. For night extension experiment, poplars grown in LD were subjected to a 4-hour dark period extension. Generation of CRISPR-Cas9 stable lines To generate CRISPR-Cas9 constructs targeting TOC1 or GI within p201N-Cas9 plasmid, specific (close to 5’-end) single guide RNA (sgRNA) were chosen from a pre-designed SNP-free dataset available on AspenDB (Supplementary Fig. 4 ) [6] , [33] . Agrobacterium tumefaciens strain GV3101/pMP90, carrying the p201N-Cas9 vector with the appropriate sgRNA, was used to transform hybrid poplar. Positive transformed poplar explants were regenerated into new plantlets [6] . 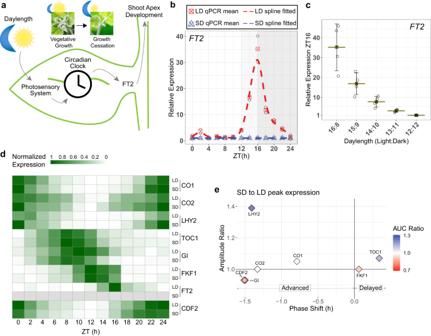Fig. 1: Daylength modulates the expression of FT2 and its transcriptional regulators to control poplar shoot apex growth. aOverview of leaf-localized daylength sensing mechanism that controls the transition from active growth to growth cessation in poplar.bDailyFT2transcription in LD (circles, red) and SD (triangles, blue). Spots represent qPCR results, with means of the two biological replicates used for fitting highlighted. Dashed lines depict a polynomial spline fit.FT2in SD was set to 1 due to nondetection.cFT2expression measured by qPCR at ZT16 under different daylengths. Mean ± sd,n= 4 biological replicates.dHeat map of daily transcription patterns for the photoperiodic-responsive genes in LD and SD. qPCR means (b and Supplementary Fig.2) normalized 0–1 per gene.FT2in SD is shown in grey due to nondetection.b–dZT, Zeitgeber Time in hours.eSD to LD deviation of the gene expression patterns shown in (d) for phase (time of maximal gene expression) shift, amplitude ratio, and daily total transcript ratio (AUC—Area Under the Curve) after Gaussian fit (Supplementary Fig.2). Genome edition was assessed by sequencing after amplifying the flanking sgRNA site using specific primers (Supplementary Table 1 ). Resulting sequences were aligned using ClustalW multiple alignment tool in the BioEdit Sequence Alignment Editor 7.0 to identify the predicted protein truncation, as indicated in Supplementary Fig. 4 [6] . Only lines showing non-functional protein predictions for both tremula and alba haplotypes were considered as positive mutants. Transient overexpression To create the TOC1 overexpressing construct, TOC1 transcript was amplified from hybrid poplar genome using the primers TOC1_FW 5’- ATGGAGGGAGAGGTAGATGAGC-3’ and TOC1_RV 5’-TTAAGATCCTGAAGCATCGTCCTCAG-3’. The resulting piece was cloned along with 35 S promoter into dpGreen destination vector using the MultiSite Gateway Kit (Invitrogen, MA, United States). Empty construct used as control was assembled in the same manner without TOC1 sequence. In vitro poplar plantlets were transformed following the protocol previously reported [34] , and leaf samples were collected after 2 days at the peak of FT2 expression. Plant phenotyping In vitro poplars were transplanted to 3.5 L pots filled with blond peat at pH 4.5 and kept under same LD growth condition. Phenotyping for the selected lines was initiated once WT plants had reached full active growth. Daylength was gradually shortened to evaluate growth cessation progression, scored from 3 (full growth) to 0 (growth absent and apical bud formed) [35] . RT-qPCR expression analysis Total RNA was extracted from young leaves of poplar plantlets using NucleoSpin RNA Plant kit (Macherey-Nagel, Düren, Germany). First-strand complementary DNA (cDNA) was synthesized using Maxima First Strand cDNA Synthesis Kit with dsDNase (Thermo Fisher Scientific, MA, United States). Quantitative real-time PCR (qPCR) analyses were carried out in a Roche LightCycler 480 II instrument (Roche Diagnostics, Barcelona, España), and values were obtained using the relative quantification method [36] . Results were relativized to UBQ7 [37] , and the log2 fold change was calculated by setting 1 the minimum expression for each gene. A list of the primers used for qPCR analysis is provided in Supplementary Table 1 . For the time course experiments qPCR data generated is provided in Supplementary Data 1 . Accession numbers Sequences of the genes called in this study can be found in Phytozome13 database with next identifiers. For poplar: CDF2 (PtXaTreH.08G068800; PtXaAlbH.08G072200), CO1 (PtXaTreH.17G090200; PtXaAlbH.17G081800), CO2 (PtXaTreH.04G088300; PtXaAlbH.04G087300), FKF1 (PtXaTreH.10G086700; PtXaAlbH.10G082000), FT2 (PtXaTreH.10G148500; PtXaTreH.10G148700; PtXaAlbH.10G142000 PtXaAlbH.10G142200), GI (PtXaTreH.05G148500; PtXaAlbH.05G150700), LHY2 (PtXaTreH.14G082800; PtXaAlbH.14G083900), and TOC1 (PtXaTreH.15G047900; PtXaAlbH.15G047900). There are 2 copies of FT2 in each haplotype derived from a local duplication [38] . For Arabidopsis : CDF2 (AT5G39660), CO (AT5G15840), FKF1 (AT1G68050), FT (AT1G65480), GI (AT1G22770), LHY (AT1G01060), and TOC1 (AT5G61380). Data-driven model of FT2 transcription The computer model was built on MATLAB_R2022a (Mathworks, Cambridge, UK). Transcriptional daily patterns of TOC1 , GI , LHY2 , and CDF2 were used as input to model the expression of FT2 under simulated light:dark cycles and mutant lines. Input patterns were fitted to a Gaussian pulse dependent of daylength. FT2 expression was defined by an Ordinary Differential Equation (ODE). A more detailed description of the methods used is provided in Supplementary Note 1 . 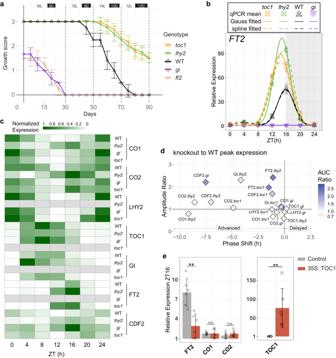Fig. 2: Circadian clock core genes TOC1, GI, and LHY2 regulate FT2 transcription. aGrowth scores from 3 (full growth) to 0 (no growth) in LD and gradually shortening the daylength, indicated by boxes on the top, for WT (black) and loss-of-function lines of TOC1 (yellow), LHY2 (green), GI (purple), and FT2 (beige)6. Mean ± sd,n= 6 biological replicates.bDailyFT2transcription in WT (upward triangles, black) compared to the knockout linestoc1(squares, yellow),lhy2(circles, green), andgi(downward triangles, purple) under LD condition. Spots depict qPCR results, with means of the two biological replicates used for fitting highlighted. Solid and dashed lines represent Gaussian and polynomial spline fits, respectively.cHeat map of daily transcription patterns for photoperiodic regulators in WT andtoc1,lhy2, andgiknockouts, under LD. qPCR means (band Supplementary Fig.5) normalized 0-1 per gene. Grey color indicates non-detection levels.dDeviation of the gene expression patterns shown in (c), comparing the respective knockout line to WT, for phase (time of maximal expression) shift, amplitude ratio, and daily total transcript ratio (AUC—Area Under the Curve).eRelative mRNA accumulation ofFT2,CO1, andCO2at ZT16 (left panel) after transiently overexpressing 35 S::TOC1 (red) or empty vector used as control (grey) in LD. Right panel shows TOC1 levels. Mean ± sd,n= 6 biological replicates. Two-sided Student’st-test, p-values from left to right: 0.0012 (**), 0.9558 (n.s.—not significant), 0.3056 (n.s.), and 0.0053 (**).b,c,eZT, Zeitgeber Time in hours. 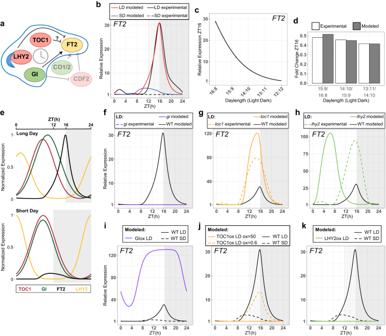Fig. 3: A minimal model that incorporates circadian regulation by TOC1, GI, and LHY2 reflects FT2 transcription dynamics under changing daylengths and genetic variations. aPhotoperiodic regulators and interactions controllingFT2expression described in poplar4,5,21. TOC1 repressive role is suggested in this work. Circadian clock genes integrated in the model are highlighted. Green and red colors denote positive and negative regulators, respectively.bSimulatedFT2transcription fit (LD-red, SD-blue) to experimental data (spline fitted; LD-black/solid, SD-black/dashed).cSimulatedFT2expression at ZT16 (peak) under different daylengths.dPredictedFT2expression fold change at ZT16 for indicated photoperiods (values inc; grey bars) compared to experimentally observed (calculated from mean values shown in Fig.1c; white bars).ePhase expression patterns of TOC1 (red), GI (green), and LHY2 (yellow) open a window forFT2transcription (black) in LD (top panel), which closes transitioning to SD to suppressFT2expression (bottom panel). Gene expression is normalized to 0-1 for visualization. Related to Supplementary Fig.8and Supplementary Movie1.f–hFT2expression predictions in simulated loss-of-function mutants for GI (f), TOC1 (g), and LHY2 (h) (solid lines) compared to experimental data (spline fitted; dashed lines) under LD. WT expression in black.i–kSimulatedFT2transcription after constitutive overexpression of GI (i), TOC1 (j), and LHY2 (k) compared to WT in LD (black/solid) and in SD (black/dashed) predictions.jFor TOC1, two levels of ectopic expression were considered. See Supplementary Note1for details. ZT, Zeitgeber Time in hours. Optimal parameters values are listed in Supplementary Table 2 . MATLAB code that allows the simulation of the model under different daylengths and genotypes scenarios can be found in Supplementary Data 2 . Reporting summary Further information on research design is available in the Nature Portfolio Reporting Summary linked to this article.